Transient expression of Bcl6 is sufficient for oncogenic function and induction of mature B-cell lymphoma Diffuse large B-cell lymphoma (DLBCL) is the most common lymphoma and can be separated into two subtypes based upon molecular features with similarities to germinal centre B-cells (GCB-like) or activated B-cells (ABC-like). Here we identify gain of 3q27.2 as being significantly associated with adverse outcome in DLBCL and linked with the ABC-like subtype. This lesion includes the BCL6 oncogene, but does not alter BCL6 transcript levels or target-gene repression. Separately, we identify expression of BCL6 in a subset of human haematopoietic stem/progenitor cells (HSPCs). We therefore hypothesize that BCL6 may act by ‘hit-and-run’ oncogenesis. We model this hit-and-run mechanism by transiently expressing Bcl6 within murine HSPCs, and find that it causes mature B-cell lymphomas that lack Bcl6 expression and target-gene repression, are transcriptionally similar to post-GCB cells, and show epigenetic changes that are conserved from HSPCs to mature B-cells. Together, these results suggest that BCL6 may function in a ‘hit-and-run’ role in lymphomagenesis. As the most common aggressive lymphoma afflicting nearly 30,000 Americans each year, diffuse large B-cell lymphoma (DLBCL) is highly heterogeneous. Current combination therapeutic regimens typically fail in nearly half of all patients with DLBCL, many of whom succumb to their disease. Given the inability to cure many patients with DLBCL, and the significant toxicity of current therapies, better treatment strategies are needed. We previously described a major molecular determinant of this biological and clinical heterogeneity, likely reflecting the cellular origin of tumours. Patients with tumours that have transcriptional profiles related to germinal centre B-cells (GCB-like) have a better overall survival than those with tumours having a transcriptional profile related to post-GCB-activated B-cells (ABC-like) [1] . This finding has been validated by several groups independently, and the molecular basis for this diversity in DLBCL has been partially deciphered in studies of distinctive genomic aberrations and somatic mutations in DLBCL subtypes. Genomic studies have defined a subset of alterations that stratify between the two DLBCL subtypes [2] , [3] , with point mutations of histone-modifying genes and B-cell receptor signalling components as the prevailing dominant drivers or accelerators of the disease [4] . However, these alterations are found in only a fraction of patients, and the relationship between more common genetic alterations and DLBCL subtypes remains largely obscure. For example, the most frequent somatic alteration observed in DLBCL, involving genetic translocation of BCL6 , is arguably the most prominent and paradoxical [5] , [6] . BCL6 is a central regulator of germinal centre development [7] , [8] ; is more highly expressed in the GCB-like subtype of DLBCL compared with the ABC-like subtype; and is associated with a favourable prognosis [1] , [9] . Yet genetic translocations of this gene are more prominent in the post-GCB subtype of the disease and are associated with adverse outcome [1] , [10] . Recent findings have implicated BCL6 in leukaemia stem cell survival [11] , [12] , and show that its activity may be altered by CREBBP or EP300 mutation [3] at an early-stage lymphoma development [13] , [14] . Separately, genetic and epigenetic aberrations in premalignant haematopoietic progenitors have recently been described in several haematological malignancies, including acute myeloid leukemia and chronic lymphocytic leukemia [15] , [16] , [17] , [18] . Together, these findings led us to postulate that BCL6 may promote tumorigenesis in a manner contrasting that of other traditional oncogenes that act in fully evolved tumour cells and require persistent activity due to oncogene addiction [19] . Somatic DNA copy number alterations (SCNAs) perturb more of the cancer genome than any other somatic alteration, and can alter the gene dosage and subsequent expression of multiple genes in a single alteration [20] . The significance of SCNAs can be assessed from the patterns of broad and focal gains/losses across the genomes of a tumour cohort, allowing potential target genes within conserved regions of DNA copy number gain/loss to be identified. The integration of expression profiling data has additionally allowed putative driver genes within each lesion to be localized by their changes in transcript abundance resulting from altered gene dosage [21] . However, a subset of oncogenes with negative feedback loops may act in a ‘hit-and-run’ fashion; therein, transient expression of the oncogene may induce broad changes to the cancer genome, epigenome or transcriptome, and be sufficient for oncogenesis in the absence of persistent expression. These ‘hit-and-run’ oncogenes may therefore not be detected by integrative analysis of DNA copy number and gene expression changes, and are difficult to identify in the absence of other genetic alterations targeting the same locus, such as genetic translocations or somatic mutations. Here we use high-resolution analysis of DNA copy number across a large cohort of DLBCL tumours to elucidate recurrent alterations in this disease. We identify gain of the BCL6 oncogene as being a potential ‘hit-and-run’ oncogene associated with poor outcome and the ABC-like DLBCL subtype. Using transgenic mouse models, we confirm that transient expression of Bcl6 is sufficient to induce aggressive mature B-cell lymphoma that appears transcriptionally similar to activated post-GCB cells. Gain of 3q27.2 is associated with inferior outcome in DLBCL Using high-resolution DNA copy number profiles of 609 DLBCL tumours analysed using the Genomic Identification of Significant Targets in Cancer (GISTIC) method, we mapped the landscape of SCNAs in this disease. We identified 22 peaks of significant DNA copy number loss (GISTIC, Q value <0.25) and 17 peaks of significant DNA copy number gain ( Fig. 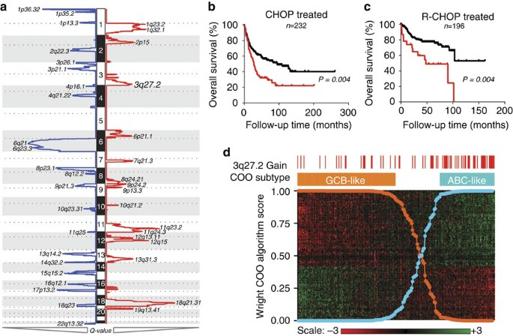Figure 1: High-resolution DNA copy number profiling of human DLBCL. (a) DNA copy number profiles from 609 primary DLBCL tumours were analysed for significant alterations using the GISTIC algorithm. This algorithm uses the magnitude and frequency of alterations at each position in the genome to assign a GISTICQvalue, with decreasing values indicating increasing significance. Significant peaks (GISTICQvalue <0.10) of DNA copy number loss (blue) and gain (red) are annotated with their genomic location. (b) In 232 patients treated with combination chemotherapy (CHOP) in the absence of Rituximab, presence of 3q27.2 gain (red) was associated with significantly worse overall survival than those with diploid copy number at this region (black). Log-rankP-value=0.004. (c) Gain of 3q27.2 (red) remained to be associated with significantly worse overall survival compared with diploid 3q27.2 (black) in 196 patients treated with combination chemotherapy plus Rituximab (R-CHOP). Log-rankP-value=0.001. (d) For 249 cases with matched gene expression profiling data, tumours were classified into GCB-like (orange) and ABC-like subtypes (blue) based upon the Wright 140 gene algorithm (heatmap shown). Gain of 3q27.2, shown by red tick marks for each case in which it was detected, was significantly over-represented in the ABC-like subtype compared with the GCB-like subtype (FisherPvalue ≤0.001). 1a and Supplementary Table 1 ). We analysed the association of each lesion with overall survival in cohorts of patients treated with combination chemotherapy (cyclophosphamide, adriamycin, vincristine, prednisone [CHOP], n =232) or in combination with Rituximab (R-CHOP, n =196). Gain of 3q27.2 was the most prognostic lesion and was associated with significantly decreased overall survival in both cohorts ( Fig. 1b,c and Supplementary Table 1 ). For 249 cases, matched gene expression profiling data was available and allowed for classification of samples into GCB-like and ABC-like subtypes using the previously defined method ( Fig. 1d ). Gain of 3q27.2 was significantly over-represented in the ABC-like DLBCL subtype (Fisher P value=8.1 × 10 −8 ), suggesting that it may contribute to the genetic aetiology of this subtype and its association with adverse outcome. Figure 1: High-resolution DNA copy number profiling of human DLBCL. ( a ) DNA copy number profiles from 609 primary DLBCL tumours were analysed for significant alterations using the GISTIC algorithm. This algorithm uses the magnitude and frequency of alterations at each position in the genome to assign a GISTIC Q value, with decreasing values indicating increasing significance. Significant peaks (GISTIC Q value <0.10) of DNA copy number loss (blue) and gain (red) are annotated with their genomic location. ( b ) In 232 patients treated with combination chemotherapy (CHOP) in the absence of Rituximab, presence of 3q27.2 gain (red) was associated with significantly worse overall survival than those with diploid copy number at this region (black). Log-rank P -value=0.004. ( c ) Gain of 3q27.2 (red) remained to be associated with significantly worse overall survival compared with diploid 3q27.2 (black) in 196 patients treated with combination chemotherapy plus Rituximab (R-CHOP). Log-rank P -value=0.001. ( d ) For 249 cases with matched gene expression profiling data, tumours were classified into GCB-like (orange) and ABC-like subtypes (blue) based upon the Wright 140 gene algorithm (heatmap shown). Gain of 3q27.2, shown by red tick marks for each case in which it was detected, was significantly over-represented in the ABC-like subtype compared with the GCB-like subtype (Fisher P value ≤0.001). Full size image The peak of this alteration (chr3:180478352-199501827) contained 134 genes, including the lymphoma oncogene BCL6 (ref. 22 ), but not a previously hypothesized target of chromosome 3 alterations, FOXP1 (ref. 23 ); Fig. 2a ). The significance of the 3q27.2 peak resulted from a combination of broad events (trisomy 3 and 3q arm-level gain) and recurrent focal gains of 3q27.2 over the BCL6 locus ( Fig. 2b ). Furthermore, 3q27.2 DNA copy number gains were mutually exclusive of translocations targeting BCL6 in the 48 tumours for which such data were available [24] , suggesting that BCL6 is a likely target of these lesions ( Fig. 2b ). However, there was no significant increase in either BCL6 expression or target gene [25] repression in cases with 3q27.2 gain compared with those cases with diploid copy number ( Fig. 2c,d ). This same trend was also observed within the context of BCL6 translocations ( Fig. 2e,f ), as previously described [10] . The absence of increased BCL6 transcript levels in tumours harbouring these genomic alterations could not be attributed to the uniformly high expression of BCL6 within DLBCL, since BCL6 transcript levels were found to be significantly lower in DLBCL than in non-malignant B-cells ( Supplementary Fig. 1 ). Together, these data led us to hypothesize that BCL6 may act in a ‘hit-and-run’ fashion and promote oncogenesis by transient overexpression during an early stage of haematopoietic differentiation or tumour evolution, and that its expression is no longer maintained or required in fully evolved tumour cells. 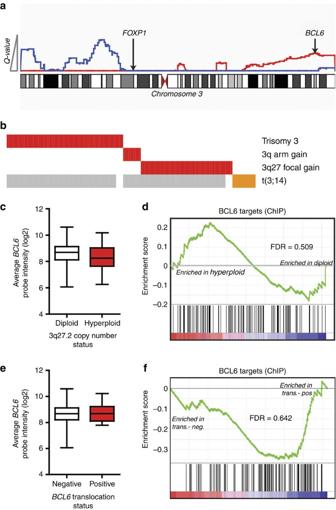Figure 2: 3q27.2 gain targetsBCL6but does not alter its expression or target-gene repression. (a) GISTICQvalues are shown for DNA copy number loss (blue) and gain (red) on chromosome 3. The peak of 3q27.2 gain included theBCL6oncogene, but not the previously described targetFOXP1. (b) Significance of 3q27.2 gain was contributed to by broad gains of chromosome 3 or the 3q arm in 76 tumours, as well as focal gains of 3q27 in 52 tumours. These gains were mutually exclusive toBCL6translocation in the 21 tumours for which matching DNA copy number and fluorescencein situhybridization data were available. Grey bars represent data not available. (c) Increased DNA copy number ofBCL6was not associated with increased transcript abundance compared with cases with no gain. Box plots represent the mean ± the interquartile range with whiskers extending to the minimum and maximum value. (d) GSEA of BCL6 target genes showed no significant repression within cases possessingBCL6DNA copy number gain (GSEA FDR =0.509). (e) For the 58 tumours with matchingBCL6translocation status and gene expression profiling data,BCL6transcript abundance was not increased in tumours withBCL6translocation compared with tumours withoutBCL6translocation. Box plots represent the mean ± the interquartile range with whiskers extending to the minimum and maximum value. (f) Tumours withBCL6translocation (Trans. pos.) showed no significant repression of BCL6 target genes by GSEA (GSEA FDR=0.642) compared with tumours withoutBCL6translocation (Trans. neg.). Figure 2: 3q27.2 gain targets BCL6 but does not alter its expression or target-gene repression. ( a ) GISTIC Q values are shown for DNA copy number loss (blue) and gain (red) on chromosome 3. The peak of 3q27.2 gain included the BCL6 oncogene, but not the previously described target FOXP1 . ( b ) Significance of 3q27.2 gain was contributed to by broad gains of chromosome 3 or the 3q arm in 76 tumours, as well as focal gains of 3q27 in 52 tumours. These gains were mutually exclusive to BCL6 translocation in the 21 tumours for which matching DNA copy number and fluorescence in situ hybridization data were available. Grey bars represent data not available. ( c ) Increased DNA copy number of BCL6 was not associated with increased transcript abundance compared with cases with no gain. Box plots represent the mean ± the interquartile range with whiskers extending to the minimum and maximum value. ( d ) GSEA of BCL6 target genes showed no significant repression within cases possessing BCL6 DNA copy number gain (GSEA FDR =0.509). ( e ) For the 58 tumours with matching BCL6 translocation status and gene expression profiling data, BCL6 transcript abundance was not increased in tumours with BCL6 translocation compared with tumours without BCL6 translocation. Box plots represent the mean ± the interquartile range with whiskers extending to the minimum and maximum value. ( f ) Tumours with BCL6 translocation (Trans. pos.) showed no significant repression of BCL6 target genes by GSEA (GSEA FDR=0.642) compared with tumours without BCL6 translocation (Trans. neg.). Full size image BCL6 expression in human haematopoietic precursors To investigate the potential for BCL6 to be acting at an early stage of haematopoietic differentiation, we performed gene expression profiling of 183 single-sorted human haematopoietic stem/progenitor cells (HSPCs) from bone marrow aspirates of two healthy adults ( Supplementary Fig. 2 ). Single-cell profiling was used in order to allow evaluation of small populations of cells possessing unique gene expression phenotypes that may not be discernible from analysis of bulk populations. Using the beta-2-microglobulin ( B2M ) gene as a reference for successful RNA amplification and gene expression microarray analysis, we observed that BCL6 transcript was detectable in 6.5% (6/92, donor 1) to 7.7% (7/91, donor 2) of single HSPCs ( Fig. 3a ). Notably, HSPCs expressing BCL6 lacked significant expression of other markers of B-cell differentiation, including PAX5 , CD19 or CD20 (MS4A1) , among others. Nonetheless, gene set enrichment analysis (GSEA) found significant repression of BCL6-bound target genes [25] within the population of cells with expressing BCL6 transcript compared with those cells not expressing BCL6 ( Fig. 3b ). Thus, in a minor subset of adult human HSPCs, BCL6 expression is associated with an early transcriptional program, consistent with similar observations in human cord blood, implicating this transcription factor in the commitment of specific progenitors to the lymphoid fate [26] . 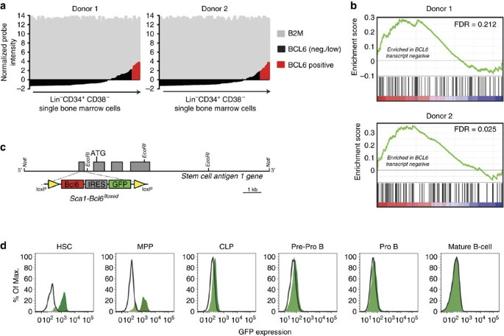Figure 3: Expression and activity ofBCL6in human and murine HSPCs. (a) Gene expression profiles of single human HSPCs showing expression of the control geneB2Mwere investigated for expression ofBCL6. Positive expression values defined as being 2 s.d.’s above the mean were observed in 11/183 single cells, with approximately equal proportions in each donor. (b) GSEA of BCL6 target genes inBCL6transcript-positive cells compared withBCL6transcript-negative cells in each donor showed an enrichment of target-gene expression inBCL6transcript-negative cells (GSEA FDRs =0.212 and 0.025 for Donor 1 and 2, respectively). This corresponds to repression of target genes inBCL6transcript-positive cells. (c) TransientBcl6expression within HSPCs was achieved by placing a floxed (yellow loxP sites)Bcl6cDNA with IRES-GFP reporter under control of the of the promoter for the HSPC-specific gene, stem cell antigen-1 (Sca1). (d) Tracking of the GFP marker forBcl6transgene expression during haematopoietic development shows expression is restricted to HSPCs and not in Pro-B or mature B-cells. Images are representative of four independent experiments. For gating schema, seeSupplementary Fig. 3. Figure 3: Expression and activity of BCL6 in human and murine HSPCs. ( a ) Gene expression profiles of single human HSPCs showing expression of the control gene B2M were investigated for expression of BCL6 . Positive expression values defined as being 2 s.d.’s above the mean were observed in 11/183 single cells, with approximately equal proportions in each donor. ( b ) GSEA of BCL6 target genes in BCL6 transcript-positive cells compared with BCL6 transcript-negative cells in each donor showed an enrichment of target-gene expression in BCL6 transcript-negative cells (GSEA FDRs =0.212 and 0.025 for Donor 1 and 2, respectively). This corresponds to repression of target genes in BCL6 transcript-positive cells. ( c ) Transient Bcl6 expression within HSPCs was achieved by placing a floxed (yellow loxP sites) Bcl6 cDNA with IRES-GFP reporter under control of the of the promoter for the HSPC-specific gene, stem cell antigen-1 ( Sca1 ). ( d ) Tracking of the GFP marker for Bcl6 transgene expression during haematopoietic development shows expression is restricted to HSPCs and not in Pro-B or mature B-cells. Images are representative of four independent experiments. For gating schema, see Supplementary Fig. 3 . Full size image We therefore hypothesized that BCL6 may contribute to lymphomagenesis at a stage of development before B-cells reach full maturity. Because BCL6 shows highly conserved patterns of expression between humans and mice [27] , we tested the hypothesis by generating a murine strain that transiently expressed Bcl6 specifically within HSPCs by placing a floxed Bcl6 cDNA with an internal ribosome entry site and enhanced green fluorescent protein (IRES-eGFP) marker under control of the promoter for the Ly6A locus encoding stem cell antigen-1 ( Sca1 ; Sca1-Bcl6 floxed ) ( Fig. 3c ; ref. 28 ). As expected, using flow cytometric analysis of the co-expressed GFP marker, we detected expression in hematopoietic stem cells (HSCs) and multipotential progenitors (MPP), with expression declining in common lymphoid progenitors (CLP) towards barely detectable expression in pre-pro-B cells and no detectable expression in pro-B cells or later stages of B-cell development ( Fig. 3d and Supplementary Fig. 3 ). Therefore, this transient expression of Bcl6 during early haematopoietic development provided a means to evaluate the potential for Bcl6 to contribute to lymphoma development via a ‘hit-and-run’ mechanism. Transient Bcl6 expression induces mature B-cell lymphoma Sca1-Bcl6 floxed mice are viable and develop normally, with a typical haematopoietic system early in post-gestational development and normal germinal centre development in response to a T-cell-dependent immunogen ( Supplementary Fig. 4 ). However, by 4 weeks of age, increased numbers of HSCs, Lin-Sca1 + c-Kit + (LSK) and lineage-restricted progenitors (Lin-CD48 + CD150 + ), and decreased numbers of common lymphoid progenitors (Lin-Sca1 + CD127 + c-Kit + ) can be detected ( Supplementary Fig. 5 ). In 8-week-old mice, we also noted changes in multiple lymphocyte compartments within the bone marrow, thymus, spleen and peripheral blood ( Supplementary Fig. 6 ). In an ageing mouse colony, Sca1-Bcl6 floxed mice exhibit significantly shortened life span compared with wild-type (WT) littermates owing to the development of B-cell lymphomas in 50% (21/42) of mice ( Fig. 4a ). These lymphomas are manifested as expanded and confluent white pulp nodules composed of pleomorphic large B-cells resulting in splenomegaly ( Fig. 4b,c ). The lymphoma cells lack Bcl6 expression but express hallmarks of B-cell identity, such as the Pax5 transcription factor ( Fig. 4d ). These results therefore provide the first indication that transient expression of the Bcl6 oncogene in HSPCs can induce aggressive malignancies of mature B-cells. 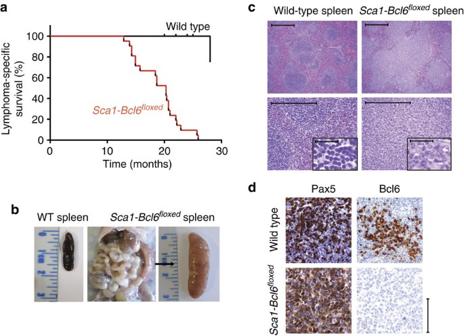Figure 4: Expression of theBcl6oncogene in haematopoietic progenitor cells (HSPCs) causes aggressive malignancy of mature B-cells that lack Bcl6 protein expression. (a) Lymphoma-specific survival ofSca1-Bcl6floxedmice (red,n=21), showing a significantly (log-rankPvalue <0.001) shortened life span compared with WT mice (black,n=20) as a result of mature B-cell malignancies. (b) Example of splenomegaly observed in 50% (21/42) ofSca1-Bcl6floxedmice. A spleen from a WT mouse is shown for reference. (c) Haematoxylin and eosin staining of WT spleens and tumour-bearing spleens fromSca1-Bcl6floxedmice shows loss of normal architecture resulting from effacement with cells morphologically resembling lymphocytes (above = × 10, below = × 40 and inset = × 400). Images are representative of ≥3 replicates. Scale bar represents 100 μm for large panels, 50 μm for inset. (d) Immunohistochemistry shows that lymphocytes fromSca1-Bcl6floxedtumours bear markers of B-cell identity (Pax5), but lack protein expression of Bcl6. WT spleens obtained from immunized mice. Scale bar represents 200 μM for all panels. Figure 4: Expression of the Bcl6 oncogene in haematopoietic progenitor cells (HSPCs) causes aggressive malignancy of mature B-cells that lack Bcl6 protein expression. ( a ) Lymphoma-specific survival of Sca1-Bcl6 floxed mice (red, n =21), showing a significantly (log-rank P value <0.001) shortened life span compared with WT mice (black, n =20) as a result of mature B-cell malignancies. ( b ) Example of splenomegaly observed in 50% (21/42) of Sca1-Bcl6 floxed mice. A spleen from a WT mouse is shown for reference. ( c ) Haematoxylin and eosin staining of WT spleens and tumour-bearing spleens from Sca1-Bcl6 floxed mice shows loss of normal architecture resulting from effacement with cells morphologically resembling lymphocytes (above = × 10, below = × 40 and inset = × 400). Images are representative of ≥3 replicates. Scale bar represents 100 μm for large panels, 50 μm for inset. ( d ) Immunohistochemistry shows that lymphocytes from Sca1-Bcl6 floxed tumours bear markers of B-cell identity (Pax5), but lack protein expression of Bcl6. WT spleens obtained from immunized mice. Scale bar represents 200 μM for all panels. Full size image Sca1-Bcl6 floxed DLBCL tumours resemble post-GCB cells We next sought to evaluate the relationship of this model with the trends observed in human DLBCL by assessing whether these malignancies resembled cells at a GCB or post-GCB (ABC/plasmablast) stage of differentiation. Using transcriptome analysis, we identified 750 significantly repressed and 720 significantly induced genes ( T -test false discovery rate (FDR) <0.25) in tumour-bearing spleens from Sca1-Bcl6 floxed mice compared with spleens from WT mice, including increased expression of multiple genes with roles in oncogenesis ( Fig. 5a and Supplementary Data 1 ). However, BCL6 target genes were not significantly repressed within these tumours (GSEA FDR=1.000; Fig. 5b ). This is consistent with our findings from human DLBCL tumours, and further supports a ‘hit-and-run’ role for Bcl6 in generating these aggressive B-cell malignancies. Human DLBCL tumours can be reliably classified into GCB-like or ABC-like subtypes by gene expression profiling [1] , and this can be achieved in murine models because of recent mapping of the transcriptional signatures of normal murine B-cell development [29] , [30] . Using the broad transcriptional signature of tumours from Sca1-Bcl6 floxed mice compared with signatures of normal stages of murine B-cell development, we found these tumours to most significantly align with the post-germinal centre ABC/plasmablast stage of differentiation (hypergeometric enrichment P value =0.028, FDR=0.017; Fig. 5c ). These changes included increased transcript abundance of the post-germinal centre transcription factors Irf4 , Prdm1 and Xbp1 ( Fig. 5d ). In addition, immunohistochemical staining of tumours from Sca1-Bcl6 floxed mice showed no staining for the GCB marker peanut agglutinin (PNA), but strong staining for Irf4 and the ABC-like DLBCL marker FoxP1 ( Fig. 5e ). These data therefore demonstrate that transient expression of the Bcl6 oncogene within HSPCs of Sca1-Bcl6 floxed mice is capable of inducing aggressive B-cell tumours that align with a differentiation stage comparable to human ABC-like DLBCL. 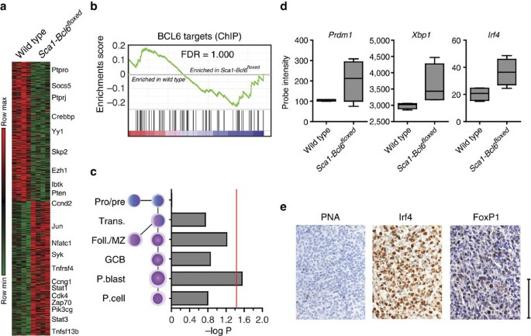Figure 5: Tumours fromSca1-Bcl6floxedmice resemble post-GCB cells. (a) Differential gene expression analysis of tumour-bearing spleens of fourSca1-Bcl6floxedmice compared with spleens from four WT mice show significant differences. These differences include genes that are involved in B-cell signalling and cell cycle regulation. (b) GSEA identified no significant repression or derepression ofBcl6target genes inSca1-Bcl6floxedtumour-bearing spleens compared with spleens from WT mice (GSEA FDR=1.000). This is in line with what is observed in human DLBCL that possess amplification of theBCL6coding region. (c) Analysis of differentially expressed genes inSca1-Bcl6floxedtumour-bearing spleens with relation to gene expression signatures of normal murine B-cell differentiation including Pro/pre-B, transitional (Trans.) B-cells, follicular and marginal zone (Foll./MZ) B-cells, GCB cells, plasmablasts (P.blast) and plasma cells (P. cell). This shows significant enrichment of the normal plasmablast signature (hypergeometric enrichmentPvalue =0.028, FDR=0.17). Red line represents a hypergeometric enrichmentPvalue of 0.05. (d) Tumours fromSca1-Bcl6floxedmice show increased expression of transcription factors that are associated with post-germinal centre stages of B-cell differentiation. Box plots represent the mean ± the interquartile range with whiskers extending to the minimum and maximum value. (e) Immunohistochemical staining shows negative expression of the germinal centre marker peanut agglutinin (PNA), but positive staining for the post-germinal centre transcription factor Irf4, and the ABC-like DLBCL marker FoxP1. Images are representative of ≥3 replicates. All panels are × 60, scale bar, 100 μm. Figure 5: Tumours from Sca1-Bcl6 floxed mice resemble post-GCB cells. ( a ) Differential gene expression analysis of tumour-bearing spleens of four Sca1-Bcl6 floxed mice compared with spleens from four WT mice show significant differences. These differences include genes that are involved in B-cell signalling and cell cycle regulation. ( b ) GSEA identified no significant repression or derepression of Bcl6 target genes in Sca1-Bcl6 floxed tumour-bearing spleens compared with spleens from WT mice (GSEA FDR=1.000). This is in line with what is observed in human DLBCL that possess amplification of the BCL6 coding region. ( c ) Analysis of differentially expressed genes in Sca1-Bcl6 floxed tumour-bearing spleens with relation to gene expression signatures of normal murine B-cell differentiation including Pro/pre-B, transitional (Trans.) B-cells, follicular and marginal zone (Foll./MZ) B-cells, GCB cells, plasmablasts (P.blast) and plasma cells (P. cell). This shows significant enrichment of the normal plasmablast signature (hypergeometric enrichment P value =0.028, FDR=0.17). Red line represents a hypergeometric enrichment P value of 0.05. ( d ) Tumours from Sca1-Bcl6 floxed mice show increased expression of transcription factors that are associated with post-germinal centre stages of B-cell differentiation. Box plots represent the mean ± the interquartile range with whiskers extending to the minimum and maximum value. ( e ) Immunohistochemical staining shows negative expression of the germinal centre marker peanut agglutinin (PNA), but positive staining for the post-germinal centre transcription factor Irf4, and the ABC-like DLBCL marker FoxP1. Images are representative of ≥3 replicates. All panels are × 60, scale bar, 100 μm. Full size image Evidence for HSPCs as lymphoma-initiating cells To exclude the potential contribution to lymphomagenesis of persistent ectopic Bcl6 expression in the mature B-cell compartment, we crossed the Sca1-Bcl6 floxed mice with an mb1-Cre mouse strain. The resulting strain, Sca1-Bcl6 Δ , maintains expression of Bcl6 under the Sca1 promoter in HSPCs, but deletes the exogenous floxed Bcl6 cDNA upon B-lineage commitment via Cre-recombinase driven by the promoter from mb1 locus encoding the immunoglobulin-associated alpha-chain Cd79a ( Fig. 6a ). To validate the efficient deletion of the exogenous floxed Bcl6 cDNA, we sorted B220 + cells from bone marrow of young Sca1-Bcl6 Δ mice and cultured under conditions to allow the isolation and expansion of a pure population of B220 + c-Kit + pro-B cells. Southern blot analysis of DNA from these cells confirmed uniform and efficient deletion of the exogenous floxed Bcl6 cDNA at the pro-B stage, and therefore all subsequent stages, of B-cell differentiation ( Fig. 6b and Supplementary Fig. 7 ). 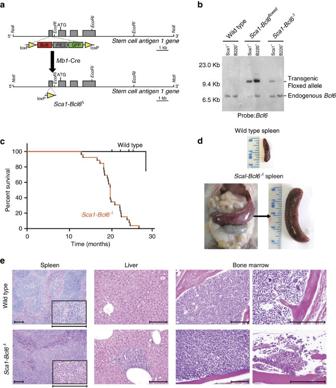Figure 6: Cre-mediated deletion of the exogenousBcl6allele in precursor B-cells does not alter formation of mature B-cell malignancies. (a) Diagramatic representation of the Sca1-Bcl6Δmice, showing expression of the transgenicBcl6allele within HSPCs under control of theSca1promoter, followed by Cre-mediated deletion at an early Pro-B cell stage uponMb1expression. (b) Southern blot analysis confirms absence of the transgenicBcl6allele within mature (B220+) B-cells ofSca1-Bcl6Δmice. Image is representative of three replicate experiments. (c) Lymphoma-specific survival ofSca1-Bcl6Δmice (n=13) demonstrates a significantly (log-rankPvalue <0.001) shorter life span compared with WT mice (n=20). (d) Example of splenomegaly observed inSca1-Bcl6Δmice, with spleen from a WT mouse is shown for reference. Images are representative of 13 mice. (e) Effacement of spleen ( × 100, inset × 400) by malignant B-cells and infiltrates in the liver ( × 200) and bone marrow (left × 200, right × 400) result in loss of normal architecture. Images representative are of 13 mice. Scale bar, 200 μm. Figure 6: Cre-mediated deletion of the exogenous Bcl6 allele in precursor B-cells does not alter formation of mature B-cell malignancies. ( a ) Diagramatic representation of the Sca1-Bcl6 Δ mice, showing expression of the transgenic Bcl6 allele within HSPCs under control of the Sca1 promoter, followed by Cre-mediated deletion at an early Pro-B cell stage upon Mb1 expression. ( b ) Southern blot analysis confirms absence of the transgenic Bcl6 allele within mature (B220 + ) B-cells of Sca1-Bcl6 Δ mice. Image is representative of three replicate experiments. ( c ) Lymphoma-specific survival of Sca1-Bcl6 Δ mice ( n =13) demonstrates a significantly (log-rank P value <0.001) shorter life span compared with WT mice ( n =20). ( d ) Example of splenomegaly observed in Sca1-Bcl6 Δ mice, with spleen from a WT mouse is shown for reference. Images are representative of 13 mice. ( e ) Effacement of spleen ( × 100, inset × 400) by malignant B-cells and infiltrates in the liver ( × 200) and bone marrow (left × 200, right × 400) result in loss of normal architecture. Images representative are of 13 mice. Scale bar, 200 μm. Full size image Importantly, Sca1-Bcl6 Δ mice recapitulate the phenotype observed in Sca1-Bcl6 floxed mice. These mice have a shortened survival compared with WT littermates ( Fig. 6c ) because of aggressive B-cell malignancy in 56.50% (13/24) of mice, manifesting as splenomegaly resulting from complete effacement of normal architecture by diffuse B-cell infiltration ( Fig. 6d,e ). Malignant B-cells are primarily immunoglobulin M (IgM + ) but show evidence of heavy-chain class-switch in a subset of tumours ( Supplementary Fig. 8 ). These mice also showed infiltration of malignant cells into the liver and bone marrow, resulting in disruption of normal architecture ( Fig. 6e ). Tumours showed increased clonality of immunoglobulin rearrangements ( Supplementary Fig. 9 ), and significant similarity to Sca1-Bcl6 floxed tumours at the transcriptional level ( Supplementary Fig. 10 ). In line with Sca1-Bcl6 floxed tumours, Sca1-Bcl6 Δ tumours also expressed markers of B-cell identity and a post-germinal centre stage of differentiation ( Supplementary Fig. 10 ). To identify the tumour repopulating cells for Sca1-Bcl6 Δ lymphomas, we purified LSK and B220 + cells and transplanted them into sublethally irradiated syngeneic recipient mice. Each of the mice transplanted with LSK cells developed a DLBCL that was phenotypically identical to the primary disease. In contrast, the B220 + cells were incapable of inducing lymphoma in secondary recipients, even when injected in a 10- or 100-fold higher number than the LSK cells ( Supplementary Table 2 ), despite these cells being able to transplant disease in other models [31] . This indicates that Bcl6 -induced DLBCL in this model is propagated by transformed HSPC cells but not mature tumour cells, and confirm that activity of the Bcl6 oncogene restricted to HSPCs can induce malignancies in mice that are of a post-germinal centre stage of differentiation. p53 loss in Sca1-Bcl6 floxed mice does not promote lymphoma Prior studies have shown that Bcl6 acts in myeloid leukaemia stem cells and normal B-cell development by inactivation of p53 and subsequent sensing of DNA damage [11] , [12] . We therefore evaluated whether the inactivation of p53 and the accumulation of secondary genetic alterations have a role in this model by crossing Sca1-Bcl6 floxed mice with heterozygous (p53 +/− ) or homozygous (p53 −/− ) p53 knockout mice. This showed that decrease or loss of p53 did not facilitate B-cell lymphoma development, but instead resulted in myeloid neoplasia ( Supplementary Fig. 11 ). B-cell lymphoma development in Sca1-Bcl6 floxed mice therefore may not proceed via suppression of p53 and the accumulation of secondary genetic lesions as observed in myeloid malignancies. Exome sequencing of Sca1-Bcl6 floxed tumours revealed the accumulation of many somatic variants, but none that were recurrent across tumours or that had been implicated in lymphomagenesis. We also noted an absence of DNA copy number abnormalities that are associated with p53 deregulation in lymphoma [32] ( Supplementary Fig. 12 and Supplementary Data 2 ). Together these data show that p53 dysfunction in combination with Bcl6 promotes myeloid malignancy, as previously described [11] . Epigenetic changes associated with transient Bcl6 expression Bcl6 mediates suppression of target genes via recruitment of factors that epigenetically modify chromatin. We hypothesized that this may elicit changes in DNA methylation, a mark that is capable of acting in gene-silencing memory [33] , and therefore investigated whether this may be a potential mechanism for Bcl6 -mediated ‘hit-and-run’ oncogenesis. Using genome-wide DNA methylation profiling by reduced representation bisulfite sequencing of populations of HSPCs and mature B-cells from WT and Sca1-Bcl6 Δ mice, we identified broad epigenetic changes associated with the expression of Bcl6 in HSPCs ( Fig. 7a and Supplementary Data 3 ). Importantly, a significant subset of these changes were found to be maintained from HSPCs to mature B-cells in Sca1-Bcl6 Δ mice, resulting in these populations being epigenetically more similar to each other than to their comparative population from WT mice ( Fig. 7a,b ). Genomic regions found to have significant changes in DNA methylation that contained a significantly higher representation of Bcl6 DNA-binding motifs compared with those regions that showed no change in DNA methylation ( Fig. 7c ), but were not significantly enriched for genes found to be bound by Bcl6 using chromatin immunoprecipitation-sequencing (ChIP-seq) analysis of mature human B-cells [25] (hypergeometric enrichment FDR=0.990). This trend was particularly notable in genes found to be hypermethylated in Sca1-Bcl6 Δ HSPCs and mature B-cells compared with their WT counterparts. Intriguingly, concordantly hypermethylated genes in HSPCs and mature B-cells from Sca1-Bcl6 Δ mice were significantly enriched for gene sets associated with murine and human stem cells and poor outcome in human DLBCL ( Fig. 7d and Supplementary Table 3 ). Although this analysis was not performed on post-GCB tumour B-cells, we suggest that these results implicate epigenetic alterations that are imparted during transient Bcl6 expression and maintained thereafter as a mechanism for Bcl6 ‘hit-and-run’ oncogenesis. 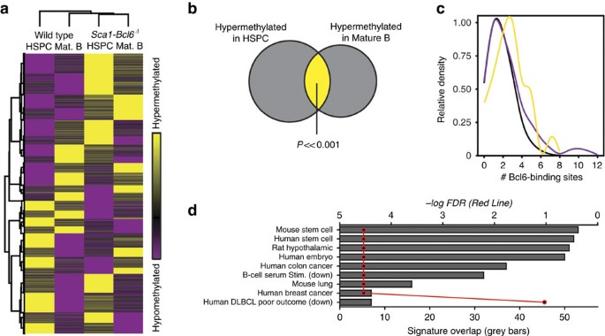Figure 7:Bcl6expression in HSPCs induced broad epigenetic changes. (a) Unsupervised hierarchical clustering of methylation ratio data from 11,258 promoter regions revealed that HSPCs and mature B-cells (Mat. B) fromSca1-Bcl6Δmice are epigenetically more similar to each other than to their respective counterparts from WT mice, again suggesting that Bcl6 acts via an epigenetic mechanism that persists from HSPCs to mature B-cells. Each condition represents a pool of biological replicates from 6 to 9 mice. (b) HSPCs and mature B-cells fromSca1-Bcl6Δmice show significant hypermethylation of a large number of genes compared with the same subsets from WT mice (Supplementary Data 3). These included a significant overlap of 470 genes, suggesting that Bcl6 creates an epigenetic signature in the HSPCs that is maintained through differentiation and can be found in the mature B-cell compartment. (c) Kernel density plot of the number of BCL6 DNA-binding sequence motifs identified in genomic regions with significant hypermehtyaltion (yellow) or hypomethylation (purple) in both HSPCs and mature B-cells fromSca1-Bcl6Δcompared with WT mice (Pvalue<0.05) and in regions with no change in methylation (black) betweenSca1-Bcl6Δand WT mice (P>0.95). Hypermethylated regions showed a significant (Pvalue <0.001) increase in the abundance of BCL6-binding motifs compared with regions with no change in methylation. Hypomethlated regions also showed a significant, but less dramatic, increase in abundance of BCL6-binding motifs (Pvalue <0.001).Pvalues calculated by Mann–WhitneyU-test. (d) Hypergeometric GSEA of the list of genes that were hypermethylated in both HSPCs and mature B-cells ofSca1-Bcl6Δmice showed significant enrichment (hypergeometric enrichment FDR <0.25) of multiple gene sets, including those associated with murine and human stem cells, and with poor outcome in DLBCL. The number of overlapping genes between those with conserved hypermethylation and those present in listed genes sets are shown by grey bars (bottomxaxis), with the corresponding FDR for the hypergeometric enrichment shown by the red line (topxaxis). Figure 7: Bcl6 expression in HSPCs induced broad epigenetic changes. ( a ) Unsupervised hierarchical clustering of methylation ratio data from 11,258 promoter regions revealed that HSPCs and mature B-cells (Mat. B) from Sca1-Bcl6 Δ mice are epigenetically more similar to each other than to their respective counterparts from WT mice, again suggesting that Bcl6 acts via an epigenetic mechanism that persists from HSPCs to mature B-cells. Each condition represents a pool of biological replicates from 6 to 9 mice. ( b ) HSPCs and mature B-cells from Sca1-Bcl6 Δ mice show significant hypermethylation of a large number of genes compared with the same subsets from WT mice ( Supplementary Data 3 ). These included a significant overlap of 470 genes, suggesting that Bcl6 creates an epigenetic signature in the HSPCs that is maintained through differentiation and can be found in the mature B-cell compartment. ( c ) Kernel density plot of the number of BCL6 DNA-binding sequence motifs identified in genomic regions with significant hypermehtyaltion (yellow) or hypomethylation (purple) in both HSPCs and mature B-cells from Sca1-Bcl6 Δ compared with WT mice ( P value<0.05) and in regions with no change in methylation (black) between Sca1-Bcl6 Δ and WT mice ( P >0.95). Hypermethylated regions showed a significant ( P value <0.001) increase in the abundance of BCL6-binding motifs compared with regions with no change in methylation. Hypomethlated regions also showed a significant, but less dramatic, increase in abundance of BCL6-binding motifs ( P value <0.001). P values calculated by Mann–Whitney U -test. ( d ) Hypergeometric GSEA of the list of genes that were hypermethylated in both HSPCs and mature B-cells of Sca1-Bcl6 Δ mice showed significant enrichment (hypergeometric enrichment FDR <0.25) of multiple gene sets, including those associated with murine and human stem cells, and with poor outcome in DLBCL. The number of overlapping genes between those with conserved hypermethylation and those present in listed genes sets are shown by grey bars (bottom x axis), with the corresponding FDR for the hypergeometric enrichment shown by the red line (top x axis). Full size image It is well established that cancer arises via the stepwise acquisition of somatic alterations that transition clones via one or more premalignant states to a malignant state [34] . But deconvolution of the stepwise events taking place during tumour cell evolution is difficult because of the many genetic alterations that become clonally dominant by the time of their interrogation within the clinically manifested tumour, and the multitude of avenues by which any given tumour can evolve. However, research within the cancer stem cell field has led to a growing appreciation for the potential of oncogenic events to be acquired by tumour cell precursors that exist at an earlier differentiation state than the evolved tumour clone [16] , [35] . Although several prior studies have implicated aberrations within HSPCs as important for driving neoplasms of mature B-cells including chronic lymphocytic leukemia [17] and follicular lymphoma [13] , [36] , there has not yet been any suggestion that a similar mechanism may be relevant for DLBCL. By high-resolution genomic analysis of a large number of human DLBCL tumours, we identified DNA copy number gain of 3q27.2 as being important for DLBCL disease biology because of its significant association with adverse outcome and the aggressive ABC-like disease subtype. Similar to many SCNAs, the minimal region of significant copy number gain on 3q27.2 contained multiple genes. However, the propensity for the BCL6 oncogene to be targeted by other genetic alterations in DLBCL, such as point mutations and translocation that deregulate its expression [24] , [6] , [37] , and the mutual exclusivity of BCL6 translocation with its DNA copy number gain, strongly suggested that BCL6 was a target of this alteration. Integrative analysis of DNA copy number and transcriptome data further suggested that BCL6 may act in a ‘hit-and-run’ fashion, wherein its transient overexpression is promoted by genetic alteration but is not maintained in the evolved tumour cell population. The BCL6 gene encodes a POZ/zinc-finger transcriptional repressor that regulates gene expression in a manner that is independent of the location of its binding site, via interaction with co-repressors that recruit histone deacetylases and induce epigenetic remodelling and heterochromatin formation [38] . The best characterized role of BCL6 is within normal B-cell activation and germinal centre formation, but its expression is not limited to the B-cell compartment and contributes to the normal function of other cellular populations, including multiple T-cell subsets and macrophages [22] , [39] , [40] , [41] , [42] . Recently, a role for BCL6 has also been described within progenitor populations during normal haematopoiesis and in the function of cancer stem cells in myeloid leukaemia [11] , [12] , [26] . Laurenti et al. [26] identified BCL6 transcript expression in human cord blood HSPCs and found that extinguishing this expression resulted in decreased numbers of mature B-cells, suggesting that Bcl6 expression in HSPCs has a critical role in early B-cell development. Our observation of BCL6 expression in a subset of adult human bone marrow HSPCs, and the associated coordinate repression of BCL6 target genes within these cells, adds to growing evidence for a role of BCL6 in normal early human haematopoiesis. It is therefore plausible that genetic deregulation of BCL6 within these cells by DNA copy number gain or translocation could potentially contribute to the pathogenesis of diseases such as leukaemia and lymphoma. The oncogenic function of BCL6 may also potentially act in the germinal centre, with repression occurring thereafter as a result of processes that occur during normal B-cell differentiation. However, transgenic mice expressing Bcl6 in mature B-cells under the control of the immunoglobulin promoter required repeated immunization in order to induce lymphoma [43] . In contrast, immunization was not required to induce lymphoma in Sca1-Bcl6 floxed or Sca1-Bcl6 Δ mice that expressed Bcl6 transiently within HSPCs, suggesting that the lymphomagenic potential of Bcl6 may be stronger within this compartment. As patterns of BCL6 expression are tightly conserved between humans and mice [27] , we modelled this hypothesis by expression of Bcl6 transiently within murine HSPCs. The lymphomas that developed in these mice were histologically similar to human DLBCL and transcriptionally similar to the differentiation stage of human ABC-like tumours in which BCL6 SCNAs were identified. Also in line with our observations in human ABC-like DLBCL, the murine lymphomas did not show overexpression of Bcl6 or coordinate target-gene repression, suggesting that Bcl6 was acting in a ‘hit-and-run’ fashion. This was further confirmed by Cre-mediated deletion of the exogenous Bcl6 allele upon B-cell maturity, which did not alter the development or phenotype of these tumours. Because BCL6 can alter the activity of the p53 tumour suppressor gene [44] , and this is critical for leukaemia stem cell survival in chronic myeloid leukaemia [12] , we investigated whether the lymphomagenic potential of transient Bcl6 expression was via repression of p53 and the accumulation of secondary genetic alterations. Crossing of Sca1-Bcl6 floxed mice with p53 +/− and p53 −/− mice did not accelerate the development of DLBCL, but instead promoted myeloid malignancies. These myeloid malignancies may have masked the development of lymphoid malignancies that have longer latency periods, but shows that combined deregulation of Bcl6 and p53 has a relatively more profound role in myeloid compared with lymphoid tumorigenesis. Furthermore, lymphomas from Sca1-Bcl6 floxed mice did not show patterns of DNA copy number change or somatic mutation that are associated with p53 malfunction in lymphoma [32] , indicating that Bcl6 may be acting ‘hit-and-run’ oncogenesis within this model in a manner that is not promoted by p53 dysfunction. Although the exact mechanism by which transient Bcl6 expression promotes oncogenesis remains to be defined, we found some evidence that suggests that Bcl6 may function by inducing epigenetic changes that were conserved from HSPCs to mature B-cells in Sca1-Bcl6 Δ mice. In addition, the reduced polyclonality of B-cell lymphomas from these mice suggested that there may be additional genetic, epigenetic or microenvironmental factors following V(D)J (Variable, Diverse and Joining gene segments) recombination that confer a growth advantage to some clones. Our observations in the mouse model described here are potentially relevant to human disease, providing some evidence for ‘hit-and-run’ oncogenesis in ABC-like DLBCLs that could be linked to BCL6 . Several lines of evidence support such a linkage. First, genetic aberrations targeting BCL6 in human DLBCL do not result in its significant overexpression or coordinate repression of its target genes. Second, we observed that genes with conserved Bcl6-induced hypermethylation between HSPC and mature B-cells of Sca1-Bcl6 Δ mice are significantly enriched for markers distinguishing human DLBCL patients with fatal/refractory disease from those that are cured. Third, correlation between DLBCL subtype and immunoglobulin heavy-chain isotype highlights an important paradox between the differentiation stage and the isotype of the B-cell receptor. Specifically, despite similar levels of activation-induced cytidine deaminase (AID) expression [10] , ABC-like DLBCL do not exhibit evidence of productive heavy-chain class-switching [45] , [46] or ongoing somatic mutation [47] . This suggests that the mature ABC phenotype of ABC-like DLBCL is disconnected from their less mature immunoglobulin genotypes. Finally, in patients presenting with relapsed/refractory disease, DLBCL subtypes exhibit differential sensitivity to salvage chemotherapy regimens as part of autologous stem and progenitor cell transplantation studies [48] , raising the hypothesis that differences in therapy might modulate BCL6 expression through epigenetic mechanisms. Although our model of ‘hit-and-run’ oncogenesis is not compatible with those genes that induce ‘oncogene-addiction’ (for example, MYC [49] ), it may be compatible with other genes that are able to induce long-lasting epigenetic changes. Whether a subset of human ABC-like DLBCL tumours have their roots in genetic aberrations arising in early HSPCs or in a more mature stem-like lymphoid subpopulation requires further study. Definitive staging of somatic genetic lesions is not obvious because tumours can exhibit phenotypes of one stage of development but contain translocations from prior stages. For example, while BCL6 , MYC , BCL2 and BCL1 translocations are all found in mature B-cell lymphomas, these lesions are distinguished by hallmarks such as immunoglobulin recombination signal sequences and junctional additions at translocation break points, suggesting their distinct derivation from early or late events during B-cell development [44] , [50] . Separately, evidence for lineage plasticity of mature lymphomas [17] , [36] complicates inferences of cell of origin that are based on either gene expression profiles or genotypes alone. It is therefore unclear as to the specific stage of haematopoietic or B-cell differentiation before evolved DLBCL that BCL6 acts, and the hierarchy of genetic events contributing to this disease will only be definitively defined by isolating human haematopoietic and tumour cell precursors from patients and identifying the minimal set of genetic lesions they harbour. Based upon our observations, we propose a model wherein an oncogene may act in a ‘hit-and-run’ fashion within early tumour cell precursors and is no longer required in the evolved tumour cell progeny. Evolved tumour cells may in turn become reliant on alternate survival pathways that are not present within their precursors. We propose that in human ABC-like DLBCL, genetic alterations of BCL6 may act in a ‘hit-and-run’ fashion in early precursors, while evolved tumour cells develop reliance on alternative oncogenic mechanisms such as nuclear-factor κB and B-cell receptor signalling pathways [51] , [52] . This may provide some explanation for the lower sensitivity of mature ABC-like DLBCL cell-lines to BCL6 inhibition [53] , despite the high prevalence of BCL6 gene alterations, and the failure of some modern targeted therapies to clear tumour stem cells, despite being effective agents against evolved tumour cells. As a consequence, targeted treatment strategies may need to be altered to accommodate combinations of agents that target oncogenic pathways that are active at both the early and late stages of tumour development. Our findings therefore have important implications for understanding and therapeutically targeting tumour cells. Integrative analysis of human DLBCL and normal B-cells All human data was obtained from public databases and associated with informed consent obtained as part of the original source studies. DNA copy number data were obtained from 609 primary DLBCL tumour specimens [23] , [32] , [54] , [55] , [56] , and were analysed by GISTIC2 (ref. 57 ). This represented all publicly available high resolution (>244,000 markers) at the time this study was undertaken. Survival annotations were available for 232 CHOP-treated patients [23] , [32] and 196 R-CHOP-treated patients [32] , [54] , as described previously. These groups of patients were analysed separately because of the improved outcome of patients treated with Rituximab. BCL6 translocation status determined by fluorescence in situ hybridization in 58 tumours with matched gene expression microarray data [24] . Raw.cel files from Affymetrix U133 plus 2.0 gene expression microarray data of 163 tumours with matched DNA copy number data and/or BCL6 translocation status [23] , [24] , [32] , and for normal B-cell subsets and DLBCL tumours [58] , were normalized by robust multi-array average (RMA) using the ExpressionFileCreator module of GenePattern [59] , and batch corrected using ComBat [60] . COO subtype was classified using the Wright algorithm of 140 genes [61] . These subtypes aligned with prior classification [23] for 125/163 cases, with the remaining discordances being transition between GCB and unclassified or ABC and unclassified, but not GCB and ABC. As a sanity check, COO was found to significantly stratify survival (log-rank P value <0.001; Supplementary Fig. 13 ). For BCL6 expression, the probe intensities of five probes specific for BCL6 were averaged (203140_at, 215990_s_at, 228758_at, 236439_at and 239249_at). Comparison of BCL6 expression between was performed using a two-sided t -test. GSEA was performed for Bcl6 target genes using a previously described set of ChIP-validated target genes [25] and GSEA-P software [62] . Single-cell gene expression profiling of human HSPCs Bone marrow from two healthy donors (1 male and 1 female) was obtained from AllCells, LLC (Emeryville, CA, USA) and sorted on a FACS ARIA II instrument as PI - , Lin - , CD34 + and CD38 - . Single cells were sorted into Terasaki plates containing alternating rows of wells containing media or Miltenyi SuperAmp lysis buffer for a total yield of 96 single cells in lysate per donor; wells containing media were visualized under a microscope to provide visual confirmation that single cells were sorted into each well ( Supplementary Fig. 2 ). For all four donors, bulk population samples were further sorted into Terasaki plates in additional groups (no further sort, HSC (CD90 + and CD45RA - ), MPP (CD90 - and CD45RA - ) and L-MPP (CD90 - and CD45RA + )), containing 200−10,000 cells. All antibodies were obtained from BD Biosciences. The lysates were shipped to Miltenyi Biotec (Auburn, CA, USA) and processed using their SuperAmp microarray service, where they amplified the lysates using their SuperAmp technology and hybridized probes made from amplified material onto SurePrint G3 Human Gene Expression 8 × 60K Microarrays (Aglient). Raw data were quantile normalized in R (Bioconductor preprocessCore library), and replicate microarray probes (representing the same gene) were log2 transformed and combined as the geometric mean. Single cells were classified as expressing BCL6 if their intensity value was 2 s.d.’s above the mean for that donor. Generation of Bcl6 transgenic mouse strains All animal work has been conducted according to relevant national and international guidelines and it has been approved by the Bioethics Committee of University of Salamanca and by the Bioethics Subcommittee of Consejo Superior de Investigaciones Cientificas (CSIC). The Bcl6-floxed vector was generated by inserting the mouse Bcl6-IRES-eGFP cassette flanked by loxP sites into the ClaI site of the pLy6 vector. The transgene fragment was excised from its vector by restriction digestion with Not I, purified and injected (2 ng ml −1 ) into CBA × C57BL/6J-fertilized eggs. Transgenic mice were identified by Southern blot analysis of tail snip DNA after Eco RI digestion, using Bcl6 cDNA to detect the transgene. Two independent transgenic lines were generated and analysed. Sca1-Bcl6 floxed mice were bred to mb1-Cre ( Cd79 atm1(cre)Reth ) mice to generate Sca1-Bcl6 Δ mice. Upon signs of disease, mice were killed and subjected to standard necropsy procedures. All major organs were examined under the dissecting microscope. Tissue samples were taken from homogenous portions of the resected organ and fixed immediately after excision. Differences in Kaplan–Meier survival plots of transgenic and WT mice were analysed using the log-rank (Mantel–Cox) test. To test the rearrangement in Sca1-Bcl6 Δ mice, different samples were analysed by Southern blot analysis after Eco RI digestion and using Bcl6 cDNA as probe. PCR was also used for confirmation, with the following primers: ClaI-F2, 5′-TATAAATCTGGCTTGATCAGG-3′ and ClaI-R2, 5′-CTGAGGAATTCATGTCTGCC-3′. Generation of Bcl6-floxed p53 −/− and Bcl6-floxed p53 +/− mice The heterozygous p53 +/− mice [63] have been described previously. Heterozygous p53 +/− mice were bred to Bcl6-floxed mice to generate compound heterozygotes. F1 animals were crossed to obtain null p53 −/− mice hemyizygous for Sca1-Bcl6 floxed mice. Tumour phenotype was assessed in the first generation of p53 heterozygous and homozygous mice. Flow cytometry Nucleated cells were obtained from total mouse bone marrow (flushing from the long bones), peripheral blood, thymus or spleen. In order to prepare cells for flow cytometry, contaminating red blood cells were lysed with red cell lysis buffer lysis buffer and the remaining cells were then washed in PBS with 1% fetal calf serum. After staining, all cells were washed once in PBS with 1% FCS containing 2 mg ml −1 propidium iodide to allow dead cells to be excluded from both analyses and sorting procedures. The samples and the data were acquired in an AccuriC6 Flow Cytometer and analysed using FlowJo software. Specific fluorescence of FITC (fluorescein isothiocyanate), PE (phycoerythrin), propidium iodide and APC (allophycocyanin) excited at 488 nm (0.4 W) and 633 nm (30 mW), respectively, as well as known forward and orthogonal light-scattering properties of mouse cells were used to establish gates. Nonspecific antibody binding was suppressed by preincubation of cells with CD16/CD32 Fc-block solution (BD Biosciences). For each analysis, a total of at least 50,000 viable (PI-) cells were assessed. The following antibodies were used for flow cytometry: anti-B220 (RA3-6B2), CD3ε (145-2C11), CD4 (RM4-5, 1:500), CD8a (53-6.7, 1:500), CD11b/Mac1 (M1/70, 1:200), CD19 (1D3), CD49b (DX5), CD117/c-Kit (2B8, 1:200), CD127/IL-7Rα (A7R34, 1:50), CD135/Flt3 (A2F10.1), Flt3 (A2B10), Ly-6G/Gr1 (RB6-8C5), IgD (11-26c.2a), IgM (R6-60.2), Sca1/Ly6A/E (E13-161.7, 1:50), CD21 (7G6), CD22 (Lyb-8.2)(Cy34.1), CD23 (B3B4), CD25 (PC61), CD48 (HM48-1), CD150 (TC15-12F12.2) and Ter119 (TER119) antibodies. Unspecific antibody binding was suppressed by preincubation with CD16/CD32 (2.4G2) Fc-block solution (Pharmingen). The different haematopoietic progenitors and B-cell stages were defined by flow cytometry as shown in Supplementary Fig. 6 . All antibodies were purchased from BD Biosciences. All antibodies were used at a 1:100 dilution unless otherwise indicated. V(D)J recombination Immunoglobulin rearrangements were amplified by PCR using the primers listed in Supplementary Table 4 (ref. 49 ). Cycling conditions consisted of an initial heat activation at 95 °C followed by 31–37 cycles of denaturation for 1 min at 95 °C, annealing for 1 min at 65 °C for heavy chains or 62 °C for light chains, and elongation for 1 min 45 s at 72 °C. This was followed by a final elongation for 10 min at 72 °C. To determine the DNA sequences of individual V(D)J rearrangements, the PCR fragments were isolated from the agarose gel and cloned into the pGEM-Teasy vector (Promega); the DNA inserts of at least 10 clones corresponding to the same PCR fragment were then sequenced. Immunohistochemistry Tissue samples were taken from homogenous portions of the resected organ by the pathologist and fixed immediately after excision. Samples of each organ were processed into paraffin, sectioned and examined histologically including routinely standard haematoxylin and eosin and immunohistochemical techniques. Transgenic mice samples were sectioned, dewaxed and heated in 10 mmol l −1 sodium citrate buffer for 30 min. Slides were incubated with primary antibodies. The antibodies used included: Bcl6 (N-3, Santa Cruz, 1:100); Pax5 (C-20, Santa Cruz, 1:125), CD21 (A-3, Santa Cruz, 1:125); and IgG (A85-I, BD Biosciences, 1:20). Samples were centrally reviewed by a panel of pathologists and diagnosed using uniform criteria based on clinical, histological, immunophenotypical and molecular characteristics. For comparative studies, age-matched mice were used. Analysis of germinal centre formation Sheep red blood cells (1–2 × 10 8 cells) were injected into the peritoneum of control, Sca1-Bcl6 floxed mice and Sca1-Bcl6 Δ mice. Ten days later, the spleens were analysed by immunohistochemistry. The spleens of control, Sca1-Bcl6 floxed mice and Sca1-Bcl6 Δ mice were isolated, embedded in OCT compound (Sakura) and snap-frozen on dry ice. Cryosections of the spleen were stained with a FITC–anti-IgD antibody (1:100 dilution, BD Biosciences) and biotinylated PNA (1:100 dilution, clone B-1075, Vector Laboratories). FITC–anti-IgD was detected with an alkaline phosphatase-coupled anti-FITC antibody (Roche), which was visualized by incubation with Fast Red (Sigma). Biotinylated PNA was detected with horseradish peroxidase-conjugated streptavidin (Zymed) followed by incubation with diaminobenzidine (Sigma). Pro-B cell culture Iscove’s modified Dulbecco’s medium supplemented with 50 μM β-mercaptoethanol, 1 mM L-glutamine, 2% heat-inactivated fetal calf serum and 0.03% (w/v) primatone RL (Sigma) was used for Pro-B cell culture experiments. Pro-B cells isolated by magnetic-activated cell sorting for B220 + (Miltenyi Biotec) from bone marrow of 2-week-old mice were cultured on irradiated ST2 cells in Iscove's Modified Dulbecco's medium containing IL-7 (R&D Systems). The cells were maintain in culture for 1 week and then collected for Southern blot experiments. Gene expression microarray analysis of murine tumours Tumour-bearing spleens were harvested from Sca1-Bcl6 floxed and Sca1-Bcl6 Δ mice, and healthy spleens were harvested from control mice; cells were not sorted before RNA extraction for this analysis. Total RNA was isolated in two steps using TRIzol (Life Technologies) followed by RNeasy Mini-Kit (Qiagen) purification following the manufacturer’s RNA Clean-up protocol with the optional On-column DNase treatment. The integrity and the quality of the RNA were verified by electrophoresis and its concentration was measured. Samples were analysed using Affymetrix Mouse Genome 430 2.0 arrays. Data were normalized as described above, and data sets containing the WT and either the Sca1-Bcl6 floxed or Sca1-Bcl6 Δ samples were filtered separately by median absolute deviation to derive the most variably expressed 10,000 genes for each comparison for use in GSEA and differential gene expression analysis. Differential gene expression analysis was performed using the ComparativeMarkerSelection module of GenePattern [59] with T -test statistic, and correcting for multiple hypothesis testing using 1,000 permutations. Genes were deemed to be significantly differentially expressed with a FDR Q value <0.25 and a fold change ≥1.25. Differentially expressed genes were tested for enrichment of genes associated with normal murine B-cell differentiation states. Gene expression signatures that are specifically upregulated in pre/pro-B cells, transitional B-cells, follicular or marginal zone B-cells, GCB cells, plasmablasts and plasma cells were assessed for their overlap with that were upregulated within tumour specimens using hypergeometric enrichment analysis [29] , [30] . The relative over abundance of a specific differentiation state within a tumour sample compared with a WT spleen is therefore detected by significant enrichment of the signature that is definitive of that differentiation state. DNA methylation profiling EpiQuest library construction : EpiQuest libraries were prepared from 200 to 500 ng mouse genomic DNA obtained from primary cells (Sca1 + Lin − cells from bone marrow, and B220 + cells and Gr1 + Mac1 + from peripheral blood) purified from Sca1-Bcl6 Δ mice and/or WT mice. DNA were pooled from 6 to 9 mice to provide one pooled replicate per condition, as performed previously [64] , [65] . The DNA was digested with 60 units of TaqI and 30 units of MspI (New England Biolabs) sequentially. Size-selected TaqI-MspI fragments (40–120 bp and 120–350 bp) were filled in and 3′-terminal-A extended, extracted with a DNA Clean & Concentrator kit (Zymo Research). Ligation to pre-annealed adaptors containing 5-methyl-cytosine (5 mC) instead of cytosine was performed using the Illumina DNA preparation kit and protocol. Purified, adaptor-ligated fragments were bisulphite-treated using the EZ DNA Methylation-Direct Kit (Zymo Research). Preparative-scale PCR (18 cycles) was performed and purified PCR products were subjected to a final size selection on a 4% NuSieve 3:1 agarose gel. SYBR-green-stained gel slices containing adaptor-ligated fragments of 130–210 bp or 210–460 bp in size were excised. Library material was recovered from the gel using a Zymoclean Gel DNA Recovery Kit (Zymo Research) and sequenced on an GAIIx genome analyzer (Illumina), yielding between 43,930,708 and 60,139,994 total reads for each condition. Sequence alignments and data analysis : Sequence reads from bisulphite-treated EpiQuest libraries were identified using standard Illumina base-calling software and then analysed using a Zymo Research proprietary computational pipeline. Residual Cs in each read were first converted to thymines (Ts), with each such conversion noted for subsequent analysis. A reference sequence database was constructed from the 36-bp ends of each computationally predicted Msp I– Taq I fragment in the 40–220-bp size range. All Cs in each fragment end were then converted to thymines. (Only the C-poor strands are sequenced in the reduced representation bisulfite sequencing process.) The converted reads were aligned to the converted reference by finding all 12-bp perfect matches and then extending to both ends of the treated read, not allowing gaps (reverse complement alignments were not considered). The number of mismatches in the induced alignment was then counted between the unconverted read and reference, ignoring cases in which a T in the unconverted read is matched to a C in the unconverted reference. For a given read, the best alignment was kept if the second-best alignment had two more mismatches; otherwise the read was discarded as non-unique. The mean CpG coverages ranged between 5-11X and total number of unique mapped reads ranged between 3,378,764 and 10,295,957 for each condition. The methylation level of each sampled C was estimated as the number of reads reporting a C, divided by the total number of reads reporting a C or T. A bioinformatics pipeline was used to score epigenetic alterations according to strength and significance, and links them to potentially affected genes. To that end, we collected a comprehensive set of regions of interest, which includes promoters, CpG islands and repetitive elements. For each of these regions, the number of methylated and unmethylated CpG observations is determined, and a P value is assigned using Fisher's exact test. Once all P values are calculated, multiple-testing correction is performed separately for each region type using the Q value method, which controls the FDR to be below a user-specified threshold (typically 10%). The software pipeline is implemented in Python (alignment processing module) and R (statistical analysis module). Unsupervised clustering was performed on methylation ratio data from each condition using Kendall tau rank correlation. Exome sequencing Next-generation sequencing libraries were prepared using NEBnext DNA sample prep kit (New England Biolabs) and exome capture performed using SureSelect XT Mouse All Exon (Agilent). Sequencing was performed using and Genome Analyzer II instrument (Illumina) with 75 bp paired-end reads, and one sample per lane. Raw sequences were trimmed by 2 bp at their 5′ ends to remove GC bias, and aligned to the murine genome (mm9) using Burrows-Wheeler Aligner with default parameters [66] . Somatic mutations and DNA copy number alterations were called with reference to age- and gender-matched controls using VarScan 2.0 (ref. 67 ). Somatic nucleotide variants were discarded if they (i) did not have a significant P value ( P ≤0.05) determined by VarScan 2.0; (ii) were not determined to be somatic alterations by VarScan 2.0; (iii) were present in ≥10% of reads within the control sample; (iv) were not observed in both strands during sequencing; and (v) were not in the coding region of a gene. Bone marrow transplantation experiments In order to determine the nature of the lymphomagenic cell, bone marrow transplantation experiments were performed. BM LSK or splenic B220 + cells were isolated and highly purified from either male Sca1-Bcl6 Δ (C57BL/6 × CBA) or male WT mice (C57BL/6 × CBA,). Mice were 12 months old. The sorting purity of these cells was analysed by FACS and determined to be over 98%. In each cohort, these cells were injected intravenously into sublethally irradiated (4 Gy) secondary recipient 12-week-old male syngenic mice (C57BL/6 × CBA). Diseased recipient mice were killed and assessed for B-cell lymphoma development. Bcl6 DNA-binding sequence motif analysis DNA sequences were obtained for genomic regions that were (i) significantly hypermethylated in both HSPCs and mature B-cells from Sca1-Bcl6 Δ mice compared with identical populations from WT mice; (ii) significantly hypomethylated in both HSPCs and mature B-cells from Sca1-Bcl6 Δ mice compared with identical populations from WT mice; and (iii) were not differentially methylated between Sca1-Bcl6 Δ mice populations and those from WT mice ( Supplementary Data 3 ). Genomic regions were searched for BCL6 DNA-binding sequence motifs (5′-TTTNNNGNNATNCTTT-3′) (ref. 68 ) using the CisFinder [69] identify motifs function, with an FDR of 0.2 and a matching threshold of 0.75. Data accession numbers: Gene expression omnibus accession number for data in this study are as follows. DNA copy number data; GSE11318 , GSE12906 , GSE15127 , GSE22082 , GSE34171 . Gene expression microarray data from from DLBCL tumors and normal B-cells; GSE11318 , GSE34171 , GSE12453 . Data produced by this study; GSE36503 , GSE56310 . How to cite this article: Green, M. R. et al. Transient expression of Bcl6 is sufficient for oncogenic function and induction of mature B-cell lymphoma. Nat. Commun. 5:3904 doi: 10.1038/ncomms4904 (2014).